Initialized near-term regional climate change prediction Climate models are seen by many to be unverifiable. However, near-term climate predictions up to 10 years into the future carried out recently with these models can be rigorously verified against observations. Near-term climate prediction is a new information tool for the climate adaptation and service communities, which often make decisions on near-term time scales, and for which the most basic information is unfortunately very scarce. The Fifth Coupled Model Intercomparison Project set of co-ordinated climate-model experiments includes a set of near-term predictions in which several modelling groups participated and whose forecast quality we illustrate here. We show that climate forecast systems have skill in predicting the Earth’s temperature at regional scales over the past 50 years and illustrate the trustworthiness of their predictions. Most of the skill can be attributed to changes in atmospheric composition, but also partly to the initialization of the predictions. Near-term climate, understood as the future climate for periods ranging between 2 and 30 years, is the combined result of a forced component due to changes in atmospheric composition, such as greenhouse gases, aerosols and other species of anthropogenic and natural origin, and an internally generated component [1] . Climate projections, which attempt to estimate the future evolution of the forced component of the climate system based on forcing scenarios, have been until recently the only source of near-term information available to the climate adaptation and mitigation communities. As an alternative, climate prediction aims at issuing statements about the future evolution of some aspect of the climate system, encompassing both forced and internally generated variations. Near-term climate prediction originated from attempts to satisfy a growing demand for climate information for the near future [2] , [3] , [4] . Slow components of the natural climate variability, associated mainly but not solely with the ocean state, can be predictable. Many of the changes in the atmospheric composition tend to have a slow pace and have delayed effects, which also induce predictability [5] . Different approaches to perform near-term climate predictions and that exploit the different sources of predictability are available. In all cases, an assessment of the forecast quality has to be made. This is achieved by performing as many predictions for the past as the available observations and computing resources permit. These predictions are expected to use only contemporaneous information available at the time of making the simulation (that is, no future information relative to the start date is used) and are known in the prediction literature as ‘hindcasts’. There have been attempts to predict near-term climate variations by exploiting empirical relationships based on past observations as well as expected physical relationships. This includes empirical models that could take into account changes in atmospheric and solar irradiance, as well as the state of the internal variability [6] , [7] , [8] . Climate projections, which are simulations with no information about the contemporaneous state of the climate system at the time of releasing the information, performed as part of the Third Coupled Model Intercomparison Project (CMIP3 (ref. 9 )) have also been used to issue climate predictions [10] , [11] , [12] . This approach did not take into account internal variability as a source of predictability. As a more ambitious approach, dynamical climate prediction explores the ability of climate models to predict regional climate changes in the near future by exploiting both initial-condition information and changes in atmospheric composition. The purpose of the initialization is to use the predictability of the internal climate variability to reduce the prediction error relative to that of the projections, whose simulations do not consider the possibility of phasing the internal variability with the observations. The extent to which this goal is achievable depends on the quality of the initial conditions, particularly of the ocean state, the quality of the climate forecast system and the initialization procedure. For the time scales ranging between a few seasons to one decade, it has been shown [2] , [3] , [4] , [13] , [14] , [15] , [16] , [17] that there is skill in near-term predictions and that the initial state can improve climate forecasts a few years ahead. However, skill improvements with the initialization appeared in disparate regions depending on the forecast system considered, the North Atlantic being a common denominator. Besides, the skill estimates were highly uncertain because of the low number of start dates considered to estimate the forecast quality. Climate predictions suffer from errors due to unavoidable uncertainties, which prevent forecast systems from taking full advantage of the large range of predictability sources. There are three main sources of uncertainty in climate prediction [18] , [19] . The first source arises from natural internal variability, intrinsic to the climate system. Internal variability could be initialized in a prediction, but the uncertainty in the initial conditions due to our inability to perfectly know the state of the climate system is non-linearly amplified. The second source is the uncertainty in the past, present and future changes in the forcing of the climate system (anthropogenic emissions, land use and natural forcings such as volcanic eruptions and solar activity) arising from a lack of observations and the limitations to know their future evolution. The third source is the uncertainty in the response of the climate system to the different external forcings. Because of the chaotic nature of the climate system and the inadequacy of current forecast systems, quantifying uncertainty has an important role in climate forecasting [20] . Dealing with uncertainty helps decision makers reach better decisions on whether or not to take any action, given the probability forecast of an event. Climate forecasting uses the ensemble method, where a set of independent forecasts with slightly different initial conditions is generated using either one or several (in the multi-model approach) dynamical forecast systems. The spread of the set of predictions represents the divergence of the solutions offered by the different forecast systems and in perfect systems is a measure of the precision of the predictions. It is expected to serve as a measure of the prediction error resulting from the three types of uncertainties, although this measure does not take account of forecast system mutual dependencies [21] , [22] . The uncertainty in near-term predictions appears to be dominated, especially on regional scales, by internal variability and model uncertainty [18] . The co-ordinated nature of the Fifth CMIP (CMIP5 (ref. 23 )) near-term ensemble prediction experiments allows, for the first time, obtaining robust estimates of the level of skill of state-of-the-art near-term climate prediction, while taking advantage of the increase in prediction reliability issued by multiple forecast systems in what is known as the multi-model approach [4] , [24] . Moreover, it offers a unique opportunity to determine to what extent the initialization improves the climate information beyond what is already provided by the traditional climate projections. This paper shows that the most comprehensive set of predictions available to date has significant skill in predicting multi-annual near-surface air-temperature averages, suggesting that climate forecast systems could have provided regional skilful information about the Earth’s climate over the past 50 years. Prediction of global and large-scale temperature indices Global-mean near-surface air temperature and the Atlantic multi-decadal variability (AMV) and the interdecadal Pacific oscillation (IPO) indices are used as benchmarks to assess the ability to predict multi-annual variability [4] , [25] ( Fig. 1 ). The AMV and IPO are the dominant decadal ocean surface temperature variations over the North Atlantic [26] and Pacific Oceans [27] , respectively, and have well-defined spatial characteristics [4] . Both indices have been estimated after removing the global-mean sea surface temperature (SST) to retain the differential cooling or warming of the corresponding basin with respect to the global behaviour. Apart from the multi-annual variability, these indices display either a long-term trend or low-frequency variability, which should be correctly predicted too. 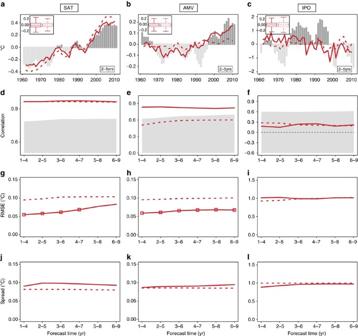Figure 1: Forecast quality of several climate indices. (a–c) Time series of the ensemble-mean forecast anomalies averaged over the forecast years 2–5 (solid, Init) and the accompanying non-initialized (dashed, NoInit) experiments of the global-mean near-surface air temperature (SAT) (a), the AMV (b) and IPO (c) indices. The observational time series, GISS49global-mean near-surface air temperature and ERSST48for the AMV and IPO, are represented with dark (positive anomalies) and light (negative anomalies) grey vertical bars, where a 4-year running mean has been applied for consistency with the time averaging of the predictions. The box-and-whisker represents the multi-model ensemble range (anomalies with respect to the multi-model ensemble mean) of Init (solid) and NoInit (dashed), where the whiskers correspond to the maximum and minimum, the box to the interquartile range and the horizontal bar to the median. The predictions have been initialized once every year over the period 1961–2006. (d–f): Correlation of the ensemble mean with the observational reference along the forecast time for 4-year averages. The one-sided 95% confidence level with at-distribution is represented in grey, where the number of degrees of freedom has been computed taking into account the autocorrelation of the observational time series, which are different for each forecast time. A two-sidedt-test (with the number of degrees of freedom computed taking into account the autocorrelation of the observational time series) for the differences between the Init and NoInit correlation found no significant results with confidence ≥90%. (g–i): RMSE of the ensemble mean along the forecast time for 4-year forecast averages. Squares are used where the Init skill is significantly better than the NoInit skill with 95% confidence using a two-sided F-test where the number of degrees of freedom takes into account the autocorrelation of the observation minus prediction time series. (j–l) Ensemble spread estimated as the s.d. of the anomalies around the multi-model ensemble mean. Figure 1: Forecast quality of several climate indices. ( a – c ) Time series of the ensemble-mean forecast anomalies averaged over the forecast years 2–5 (solid, Init) and the accompanying non-initialized (dashed, NoInit) experiments of the global-mean near-surface air temperature (SAT) ( a ), the AMV ( b ) and IPO ( c ) indices. The observational time series, GISS [49] global-mean near-surface air temperature and ERSST [48] for the AMV and IPO, are represented with dark (positive anomalies) and light (negative anomalies) grey vertical bars, where a 4-year running mean has been applied for consistency with the time averaging of the predictions. The box-and-whisker represents the multi-model ensemble range (anomalies with respect to the multi-model ensemble mean) of Init (solid) and NoInit (dashed), where the whiskers correspond to the maximum and minimum, the box to the interquartile range and the horizontal bar to the median. The predictions have been initialized once every year over the period 1961–2006. ( d – f ): Correlation of the ensemble mean with the observational reference along the forecast time for 4-year averages. The one-sided 95% confidence level with a t -distribution is represented in grey, where the number of degrees of freedom has been computed taking into account the autocorrelation of the observational time series, which are different for each forecast time. A two-sided t -test (with the number of degrees of freedom computed taking into account the autocorrelation of the observational time series) for the differences between the Init and NoInit correlation found no significant results with confidence ≥90%. ( g – i ): RMSE of the ensemble mean along the forecast time for 4-year forecast averages. Squares are used where the Init skill is significantly better than the NoInit skill with 95% confidence using a two-sided F-test where the number of degrees of freedom takes into account the autocorrelation of the observation minus prediction time series. ( j – l ) Ensemble spread estimated as the s.d. of the anomalies around the multi-model ensemble mean. Full size image Non-initialized (NoInit henceforth) predictions of the global-mean near-surface air temperature are statistically significantly skilful for most of the forecast ranges as the dashed line corresponding to the ensemble-mean correlation with the observations is above the grey area in Fig. 1 . The skill in this figure is obtained as follows. For a given 4-year average forecast period, like the average of the first 4 years (years 1–4), both the multi-model ensemble mean and the observational average for the corresponding calendar dates (the years 1961 to 1964 for the 1961 start date) are collected in a time series that contains one value for each start date from 1961 to 2006. It is between these time series that the skill measure is computed. The same operation is carried out for the next 4-year average forecast period, which in the case of the 2–5-year average involves averaged values for the years 1962 to 1965 for the 1961 start date (2007 to 2010 for the 2006 start date), until the last 4-year forecast period that can be constructed with the CMIP5 10-year hindcasts, the 6–9 forecast time average. The high skill is due to the almost monotonic increase in near-surface air temperature correctly reproduced by the multi-model ensemble mean (in spite of an overestimation of the positive trend), pointing at the large role played by the time-varying radiative forcing [4] , [28] . The high correlation, although not statistically significant, of the NoInit AMV predictions all along the forecast time is also consistent with the role attributed to the external forcings in determining its recent variability [29] , although some predictability sources missing in many of the individual forecast systems considered here might also contribute to the skill in future systems [30] . Prescribed changes in the atmospheric composition, either of natural or anthropogenic origin, are the only explanation for the positive skill of the NoInit global-mean near-surface air temperature and AMV predictions, and imply that atmospheric composition changes alone would have provided skilful global-mean and non-trivial North Atlantic temperature information up to 10 years into the future over the past 50 years. The skill of these two time series improves substantially with initialization for all forecast ranges ( Fig. 1 ). The positive impact of the initialization is more obvious in terms of the ensemble-mean root mean square error (RMSE) than with the correlation when comparing the initialized (Init henceforth) with the NoInit forecast quality. The reason is that the correlation is a measure of skill that is not sensitive to errors in the linear trend [31] . The initialization can, in addition to providing information about the phase of the internal variability, correct systematic errors in the model response to external forcings [29] , [32] . An example of this correction can be seen in the time series of the global-mean near-surface air temperature, where both multi-model ensembles, Init and NoInit, reproduce the observed long-term upward trend and the largest excursions from this trend, while NoInit overestimates the trend. In contrast to the correlation, the RMSE integrates the errors linked to both the long-term trend and the internal variability, reflecting the better representation of the trend in Init. This result supports the conclusion from pioneering near-term prediction exercises [2] . In addition to a mean improvement, Fig. 1 also shows that the initialization provides more realistic predictions of the recent global-mean temperature hiatus of the early XXI Century [33] , as already suggested in Smith [34] and Meehl and Teng [35] . The IPO predictions have a positive correlation but, in sharp contrast to the global-mean near-surface air temperature and the AMV, they do not show statistically significant correlations along the forecast range, even when initialized. The Pacific, and in particular the northern part of the basin, is one of the regions with the lowest temperature skill [36] . However, the analysis of some case studies shows improved predictions for large climate fluctuations of the IPO compared with the NoInit simulations [35] . Reliability of the predicted indices Apart from the different aspects associated with forecast accuracy, users need also estimates of how reliable (i.e., whether the forecast uncertainty estimate is accurate) the predictions are [19] . Reliable (i.e., trustworthy) predictions in a perfect system typically correspond to those where the time-mean ensemble spread about the ensemble-mean prediction equals the time-mean RMSE of the ensemble-mean forecast [37] . In ensemble forecasting, the ensemble spread is used as an estimate of the prediction uncertainty. Spread estimates give more precision when using multiple forecast systems [24] , [38] . Figure 1 shows that the spread of the three indices considered does not change substantially with forecast time, in spite of increasing slowly in two of the cases. This early saturation of the spread suggests that the perturbations used to generate the ensemble only excite relatively short-term processes, which produce a mean spread that does not grow with forecast time as the mean error does [39] , and leads to the spread not being an adequate measure of the prediction precision and an inappropriate estimator of the forecast uncertainty [31] . The initialization affects the mean spread of the predictions. The spread tends to be larger for Init than for NoInit, a consequence of several individual forecast systems showing an increased spread in Init with respect to NoInit. Figure 1 shows that the Init experiment overestimates the spread for the global-mean near-surface air temperature and AMV indices, as it is larger than the RMSE, whereas NoInit underestimates the spread slightly. The spread seems to be adequate for the IPO. The Init overestimation is a particularly relevant aspect for the users of the climate information based on decadal predictions that should be carefully considered in the next generation of climate forecast systems. Regional predictions Although simple indices help to characterize the behaviour of a system, the users of climate information also require spatial information. Near-term climate forecast systems have positive near-surface temperature skill, as measured with the root mean square skill score (RMSSS) (see Methods), over large regions, which is often statistically significantly different from zero as reflected in the large stippled areas found in Fig. 2 both over the ocean and the land [3] , [4] , [17] , [24] . The regions with high skill agree in many cases with those where the relative importance of the linear trend with respect to the interannual variability is at its highest ( Fig. 3 ), which again points at the important role of the specified variations in atmospheric composition that are responsible of the upward trend in the last 50 years. 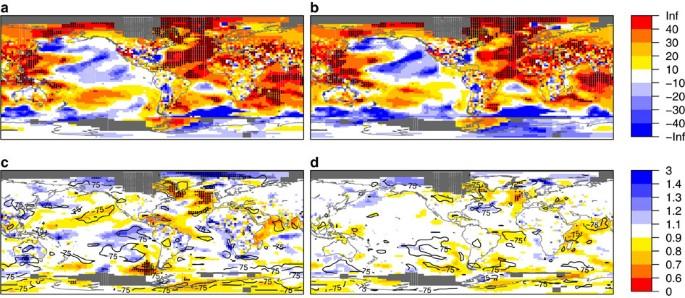Figure 2: Near-surface air-temperature forecast quality. (a,b) RMSSS (multiplied by 100) of the ensemble mean of the Init multi-model for predictions averaged over the forecast years 2–5 (a) and 6–9 (b). A combination of temperatures from GHCN/CAMS47air temperature over land, ERSST48and GISTEMP 1200 (ref.49) over the polar areas is used as a reference. Black dots correspond to the points where the skill score is statistically significant with 95% confidence using a one-sided F-test taking into account the autocorrelation of the observation minus prediction time series. (c,d) Ratio of RMSEs between the Init and NoInit multi-model experiments for predictions averaged over the forecast years 2–5 (c) and 6–9 (d). Contours are used for areas where the ratio of at least 75% of the individual forecast systems has a value above or below 1 in agreement with the multi-model ensemble-mean result. Dots are used for the points where the ratio is statistically significantly above or below 1 with 90% confidence using a two-sided F-test that takes into account the autocorrelation of the observation minus prediction time series. Poorly observationally sampled areas are masked in grey. Figure 2: Near-surface air-temperature forecast quality. ( a , b ) RMSSS (multiplied by 100) of the ensemble mean of the Init multi-model for predictions averaged over the forecast years 2–5 ( a ) and 6–9 ( b ). A combination of temperatures from GHCN/CAMS [47] air temperature over land, ERSST [48] and GISTEMP 1200 (ref. 49 ) over the polar areas is used as a reference. Black dots correspond to the points where the skill score is statistically significant with 95% confidence using a one-sided F-test taking into account the autocorrelation of the observation minus prediction time series. ( c , d ) Ratio of RMSEs between the Init and NoInit multi-model experiments for predictions averaged over the forecast years 2–5 ( c ) and 6–9 ( d ). Contours are used for areas where the ratio of at least 75% of the individual forecast systems has a value above or below 1 in agreement with the multi-model ensemble-mean result. Dots are used for the points where the ratio is statistically significantly above or below 1 with 90% confidence using a two-sided F-test that takes into account the autocorrelation of the observation minus prediction time series. Poorly observationally sampled areas are masked in grey. 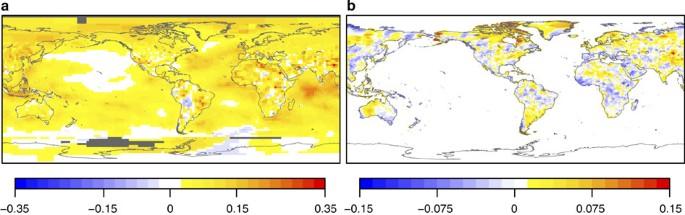Figure 3: Near-surface temperature and precipitation relative linear trends. Ratio between the slope of the linear trend and the residual variability (1 per year) over 1961–2010 for (a) near-surface temperature and (b) GPCC50precipitation. A combination of temperatures from GHCN/CAMS air temperature over land47, ERSST48and GISTEMP 1200 over the polar areas49is used as a reference. Monthly values have been smoothed with a 4-year running average before estimating the trend and the residual variance. Poorly observationally sampled areas are masked in grey. Full size image Figure 3: Near-surface temperature and precipitation relative linear trends. Ratio between the slope of the linear trend and the residual variability (1 per year) over 1961–2010 for ( a ) near-surface temperature and ( b ) GPCC [50] precipitation. A combination of temperatures from GHCN/CAMS air temperature over land [47] , ERSST [48] and GISTEMP 1200 over the polar areas [49] is used as a reference. Monthly values have been smoothed with a 4-year running average before estimating the trend and the residual variance. Poorly observationally sampled areas are masked in grey. Full size image The skill improvement due to the initialization has been assessed by computing the ratio of the RMSE of Init and NoInit. The areas in yellow and orange in Fig. 2 correspond to those points where the Init RMSE is lower, i.e., the information is more skilful, than the NoInit RMSE. The robust skill increase due to the initialization ( Fig. 2 , lower panels) is limited to areas of the North Atlantic, in agreement with previous results [3] , [13] , [16] , the southeast Pacific and the Indian Ocean. Some areas of the Southern Ocean and Antarctica also show a skill improvement with the initialization, but long-term observations are not trustworthy there and the skill, even after initialization, is still low. Robustness of the skill increase has been assessed either as the agreement in skill improvement between the individual systems or after applying a statistical inference test (see Methods). No improvements are found over land, although a different skill measure (ensemble-mean correlation) offered a positive impact of the initialization on the Mediterranean and northern Eurasia. In fact, the skill varies slightly depending on the forecast quality measure used. The improvements discussed in certain areas, like over the northern Indian Ocean, are not found when using correlation. This is because the positive impact of the initialization might be, as already mentioned for the global-mean near-surface air temperature, due to the correction of the modelled climate response induced by the initialization. Although there seems to be a predominance of areas in Fig. 2 where the Init skill is better than the NoInit skill (especially for the 2–5-year forecast time) in some regions of the subtropical Pacific, the North Atlantic and the tropical Indian Ocean, the impact of the initialization on the skill is small. The linear trend is prominent compared with the interannual variability in some of these regions ( Fig. 3 ), which reduces the effective sample size. The effect of the small sample size and the low amplitude of the differences are at the origin of the lack of statistically significant differences between Init and NoInit with 90% confidence. Although some individual forecast systems show (as documented in several publications) skill improvements with the initialization larger than the improvements reported in this article the locations where the skill differences between the Init and NoInit experiments of the individual systems are found differ widely among those systems. This is reflected in Fig. 2 in the small fraction of areas where the skill improvement with initialization of more than 75% of the systems agrees with the multi-model result. This additional measure of robustness limits the confidence on the positive impact of the initialization obtained from individual systems although still justifies the use in climate services [40] and adaptation [41] studies of the multi-model climate information described here. The Pacific Ocean is the basin with the lowest skill overall ( Fig. 2 ), with no consistent impact of the initialization. The complex basin-wide structure of the forecast quality explains the low IPO ensemble-mean skill ( Fig. 1 ). The central North Pacific has zero or negative skill, which is linked to the relatively low importance of the predictable linear trend ( Fig. 3 ), the failure in predicting the largest warming events [36] and the different behaviour of surface temperature and upper ocean heat-content predictions for the Pacific Decadal Oscillation [15] , [16] , [42] . The west subtropical Pacific, instead, has positive skill in agreement with previous results [43] . The skill for land precipitation ( Fig. 4 ) is much lower than the skill for near-surface temperature, with several regions, especially in the Northern Hemisphere, displaying positive values. However, the existence of almost as many areas around the planet with negative as regions with positive skill suggests that near-term precipitation information should be used with great caution. The most that can be done at this early stage is to try to understand the sources of the positive precipitation skill. The skill in areas like Europe and Sahelian Africa might be linked to the positive AMV skill, the AMV being a good descriptor of the multi-annual precipitation variability over those regions [4] . In other areas, like the Asian continent and the Arctic, positive skill coincides with the regions where the relative importance of the linear trend to the interannual variability is the highest ( Fig. 3 ). The positive precipitation skill can be attributed mostly to the specification of the atmospheric concentration variations as the initialization does not substantially improve the skill ( Fig. 4 , lower panels). 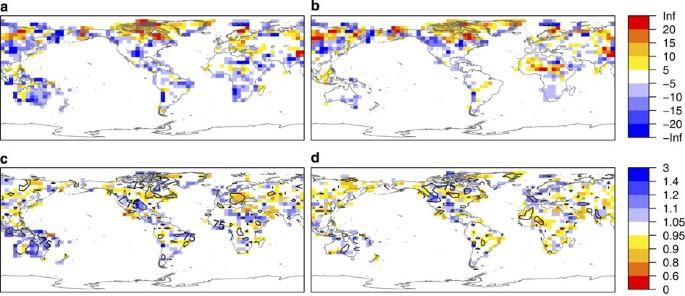Figure 4: Precipitation forecast quality. (a,b) RMSSS (multiplied by 100) of the ensemble mean of the Init multi-model for predictions averaged over forecast years 2–5 (a) and 6–9 (b). GPCC50precipitation is used as a reference. Black dots correspond to the points where the skill score is statistically significant with 95% confidence using a one-sided F-test taking into account the autocorrelation of the observation minus prediction time series. (c,d) Ratio of RMSEs between the Init and NoInit multi-model experiments for predictions averaged over forecast years 2–5 (c) and 6–9 (d). Contours are used for areas where the ratio of at least 75% of the individual forecast systems has a value above or below 1 in agreement with the multi-model ensemble-mean result. An inference tests at the grid point level was applied to assess if the ratio is statistically significantly above or below 1 with 90% confidence using a two-sided F-test that takes into account the autocorrelation of the observation minus prediction time series, but no point was found significant. Both predictions and the observational reference were smoothed to a 5° grid to reduce the spatial variability of the results. Figure 4: Precipitation forecast quality. ( a , b ) RMSSS (multiplied by 100) of the ensemble mean of the Init multi-model for predictions averaged over forecast years 2–5 ( a ) and 6–9 ( b ). GPCC [50] precipitation is used as a reference. Black dots correspond to the points where the skill score is statistically significant with 95% confidence using a one-sided F-test taking into account the autocorrelation of the observation minus prediction time series. ( c , d ) Ratio of RMSEs between the Init and NoInit multi-model experiments for predictions averaged over forecast years 2–5 ( c ) and 6–9 ( d ). Contours are used for areas where the ratio of at least 75% of the individual forecast systems has a value above or below 1 in agreement with the multi-model ensemble-mean result. An inference tests at the grid point level was applied to assess if the ratio is statistically significantly above or below 1 with 90% confidence using a two-sided F-test that takes into account the autocorrelation of the observation minus prediction time series, but no point was found significant. Both predictions and the observational reference were smoothed to a 5° grid to reduce the spatial variability of the results. Full size image More than six individual forecast systems have provided near-term hindcasts to the CMIP5 experiment, but the hindcasts were produced using the core experimental set up where only one prediction was started every 5 years, resulting in 10 predictions over the period 1961–2006 instead of 46 as used in the results shown here. As it is difficult to obtain robust forecast quality estimates with such limited samples [25] , [44] , this paper only discusses results from those systems with a higher frequency of start dates. However, a systematic comparison of the results with both samples suggests that a 5-year interval sampling allows estimating the level of skill, although the estimates contain spurious maxima along the forecast time due to the poor sampling of the start dates [25] . Users are encouraged to access predictions from multi-model forecast systems that make simulations with a 5-year interval sampling between start dates, although they should bear in mind the importance of measuring the robustness of the corresponding forecast quality estimates. Reliability of the regional predictions The spatial distribution of the spread shows that the CMIP5 multi-model overestimates the temperature spread ( Fig. 5 ) over the North Atlantic and the Arctic, and underestimates it over the North Pacific and most continental areas, both for Init and NoInit. The spread overestimation agrees with the results found for the indices in Fig. 1 and has not been thoroughly documented to date. Sufficiently reliable predictions, which require a calibrated ensemble spread, can be made taking into account the systematic errors in the model variability in a sort of calibration a posteriori [45] . However, the calibration a priori of the ensemble is more desirable than a post-processing of the predictions. This is an aspect that requires careful attention in the implementation of multi-model operational systems such as the ones that are currently planned [34] to satisfy the reliability requirements of the climate services and climate adaptation communities. 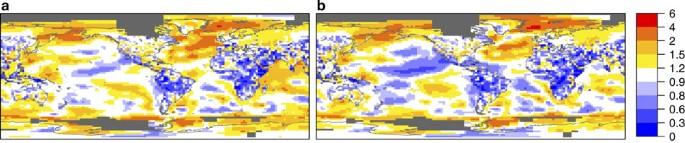Figure 5: Multi-model ensemble spread for the near-surface temperature. Ratio between the spread and the RMSE of the ensemble mean for Init (a) and NoInit (b) for the predictions averaged over forecast years 2–5. A combination of temperatures from GHCN/CAMS47air temperature over land, ERSST48and GISTEMP 1200 (ref.49) over the polar areas is used as a reference. Figure 5: Multi-model ensemble spread for the near-surface temperature. Ratio between the spread and the RMSE of the ensemble mean for Init ( a ) and NoInit ( b ) for the predictions averaged over forecast years 2–5. A combination of temperatures from GHCN/CAMS [47] air temperature over land, ERSST [48] and GISTEMP 1200 (ref. 49 ) over the polar areas is used as a reference. Full size image These results confirm that there is substantial skill in predictions of multi-annual averages of near-surface temperature when using the most comprehensive set of near-term climate predictions available to date. They suggest that climate forecast systems could have provided regional skilful information about the Earth’s climate over the past 50 years and encourages users of near-term climate information to explore the usefulness of this very innovative tool. Most of the skill is due to the slowly varying changes in atmospheric composition, both natural and anthropogenic, while the initialization of the forecast systems robustly improves several aspects of the forecast quality of global-mean near-surface air temperature and temperature over the North Atlantic and a handful of other regions. Current forecast systems also show an important overestimation of the ensemble spread, especially in skilful areas, and an underestimation for near-surface temperature in other regions. The spread overestimation points to the urgent need of a careful development of improved forecast systems that produce ensemble predictions leading to reliable, while skilful, near-term climate information for climate adaptation and services. This is already being considered in the development of near-term climate predictions in real time [34] , which would benefit from the feedback of an increasing number of users of this rapidly evolving source of climate information. Near-term prediction experiments The recognition that near-term climate prediction is important motivated the research community to design co-ordinated experiments. The ENSEMBLES project [4] , [25] conducted a multi-forecast system decadal hindcast experiment that served as inspiration to the CMIP5 near-term co-ordinated experiment [23] . To address the key uncertainties at the source of near-term forecast error, such as uncertainties in the initial conditions and associated with the model inadequacy [46] , ensemble methods have been proposed. They involve not only using a single system several times with slightly different initial conditions but also employing multi-model or perturbed-parameter approaches. In the CMIP5 near-term prediction experiments, a set of individual forecast systems performed a series of 10-year hindcasts initialized from observations every 5 years starting near the end of 1960 until the last start date at the end of 2005. To obtain robust estimates of the forecast quality, some institutions performed simulations starting once per year instead of once every 5 years. Only a subset of the institutions contributing to CMIP5 followed this practice as the computational requirements for such an experiment are prohibitive. As each individual forecast system starts at a different time near the end of the previous year, all predictions are considered to start at the beginning of each calendar year over the period 1961–2006. Because the practice of near-term prediction is in its infancy, details of how to initialize the models were left to the discretion of the modelling groups. The sample is limited by the length of the period over which reasonably accurate estimates of the ocean initial state can be made, which starts shortly before 1960. The impact of the initialization has been assessed by comparing the forecast quality of the initialized predictions with estimates of the forecast quality of a multi-model ensemble that has no information about the contemporaneous state of the climate system, which are the simulations referred to as non-initialized. The non-initialized ensemble consists in the historical, up to 2005, and the representative concentration pathways 4.5 (RCP4.5) simulations [23] , after 2006, which are sliced in 10-year chunks over the same calendar dates as the initialized hindcasts. The initialized and non-initialized ensembles are referred to as Init and NoInit, respectively, and were performed using exactly the same climate models and natural and anthropogenic forcings. Atmospheric composition, including volcanic aerosol, and solar irradiance variability were prescribed along the integration using actual values up to 2005. After that date, the RCP4.5 scenario was assumed, as well as a background solar irradiance level and a constant volcanic aerosol load. The specification of the volcanic aerosol load and the solar irradiance in the hindcasts gives an optimistic estimate of the forecast quality with respect to an operational forecast system that would use projections for these forcings. The individual forecast systems contributing to the CMIP5 multi-model are described in Table 1 . Six individual systems, which are the ones used in this paper, performed predictions started once per year instead of every 5 years. Table 1 Forecast systems contributing to the CMIP5 multi-model. Full size table Computation of the anomalies When initialized with states close to the observations in what is known as full-field initialization, models drift towards their preferred imperfect climatology, reflecting systematic errors (i.e., the difference in the climate estimates of the predictions and the observational reference) in the predictions. This drift depends on the forecast time. Forecast quality estimates have been computed using forecast and observational anomalies that take into account the systematic error of the forecast systems. Forecast anomalies have been estimated by removing the mean model climate for the specific forecast period using only the predictions for which there are observational reference data available [25] . For instance, to obtain the anomalies of the average 6–9-year forecast period from the simulations initialized in November 1970, the model climate is estimated by averaging the data for the 6–9-year forecast period from all the simulations for which there is reference data. This implies that, when using predictions started every year, data from those starting between 1961 and 2003 (44 start dates) are used, because no full reference data for the period 2012–2015 (i.e., the verifying dates of the predictions started in 2004, 2005 and 2006) are available yet. The anomalies for the reference data set are estimated for the same calendar period, but using the observational climatology. This linear method assumes that there is no relationship between the model drift and the anomalies. The same method has been used for the hindcasts produced with systems based on the anomaly-initialization method because there is no guarantee that such method completely prevents model drift. Climate indices The global-mean near-surface air temperature has been computed using an area-weighted average of the data on a regular grid. The AMV index was estimated as the SST anomalies averaged over the region Equator −60 °N and 80 °–0 °W minus the SST anomalies averaged over 60 °S–60 °N [26] . The IPO index is the principal component of the leading empirical orthogonal function (EOF) of the covariance matrix [27] (the use of the correlation matrix gave similar results) using 4-year averaged data. The EOFs were estimated for each individual forecast system using SST in the region 50 °S–50 °N/100–290 °E, where the mean SST over 60 °S–60 °N have been previously removed [4] . As the predicted EOFs might have different features to those found in the observational IPO, the spatial patterns have been visually inspected for each individual forecast system to avoid using an index that could be identified as a different mode of variability. Both the AMV and the IPO have very well-defined spatial characteristics that reflect their large-scale nature. Reference data and forecast quality assessment Different data sets have been used as reference to estimate the forecast quality. To verify near-surface temperature, a merged data set using land air temperatures from the GHCN/CAMS data set [47] and SST from the NCDC ERSST V3b data set [48] , while outside the band between 60 °N and 60 °S, the GISSTEMP data set with 1,200 km decorrelation scale was used [49] . The Global Precipitation Climatology Centre (GPCC) v5 (ref. 50 ) data set was used for precipitation. Various measures of forecast quality have been used to assess the experiments as different measures give different information about the multi-faceted forecast quality [51] . The measures include the correlation coefficient, the RMSE and the RMSSS of the ensemble mean. The RMSSS is estimated as one minus the ratio of the RMSE of the ensemble-mean prediction over the RMSE of the mean climate. The multi-model ensemble mean has been built as the average of the ensemble means of the individual forecast systems to give them the same weight in the multi-model regardless of their ensemble size. Figure 1 illustrates that skill measures can give slightly different messages, such as the large improvement in global-mean near-surface air temperature due to the initialization in terms of RMSE in contrast with the almost-negligible improvement in terms of correlation. The main reason for this is that the correlation coefficient is not sensitive to a scaling factor, so that a system that reproduces the observation but with a reduced amplitude gives a high correlation coefficient but might not give good results using other scores like the RMSE. The statistical significance for the correlation is assessed with a one-tailed t -test. The test for statistically significant differences in correlation between the initialized and non-initialized experiments is performed by employing a two-tailed t -test after a Fisher’s Z transformation. The RMSSS is tested for statistical significance (with an alternative hypothesis of RMSSS >0) using a one-tailed F-test, whereas the ratio in RMSE between the initialized and non-initialized experiments has been tested with a two-tailed F-test. An effective sample size is used in all the inference tests to avoid obtaining too liberal confidence levels. This is tackled by estimating the effective sample size as described in von Storch and Zwiers [52] . This approach takes into account the autocorrelation of the corresponding observational time series in the case of the correlation and of the differences between observations and predictions for the RMSE. As the autocorrelation function and the availability of data depends on the forecast period considered, different effective sample sizes and, hence, different confidence intervals are obtained for each forecast period, which prevents the grey shading in Fig. 1 from following a straight line along the forecast time. How to cite this article: Doblas-Reyes, F. J. et al . Initialized near-term regional climate change prediction. Nat. Commun. 4:1715 doi: 10.1038/ncomms2704 (2013).